Naturally occurring tumours in the basal metazoanHydra The molecular nature of tumours is well studied in vertebrates, although their evolutionary origin remains unknown. In particular, there is no evidence for naturally occurring tumours in pre-bilaterian animals, such as sponges and cnidarians. This is somewhat surprising given that recent computational studies have predicted that most metazoans might be prone to develop tumours. Here we provide first evidence for naturally occurring tumours in two species of Hydra . Histological, cellular and molecular data reveal that these tumours are transplantable and might originate by differentiation arrest of female gametes. Growth of tumour cells is independent from the cellular environment. Tumour-bearing polyps have significantly reduced fitness. In addition, Hydra tumours show a greatly altered transcriptome that mimics expression shifts in vertebrate cancers. Therefore, this study shows that spontaneous tumours have deep evolutionary roots and that early branching animals may be informative in revealing the fundamental mechanisms of tumorigenesis. A tumour is an abnormal growth of body tissue, which can be malignant or benign. According to Hanahan and Weinberg [1] , malignant tumours in humans should have eight characteristic properties. In invertebrates, such as flies and worms, bona fide tumours were discovered in several organ systems [2] . However, no systematic studies on the incidence of tumours in invertebrates have been undertaken up to now [3] . In particular, although there are occasional reports of growth abnormalities in sponges and cnidarians [3] , [4] , and there is a striking example of transgenically induced neoplasia in Hydractinia [5] , there are no detailed reports of spontaneous tumours outside the bilaterian clade ( Fig. 1 ). This is surprising as we have previously shown by using a phylostratigraphic approach [6] that the origin of multicellularity in animals coincides with the evolutionary emergence of genes known to be involved in human cancer formation ( Fig. 1 ). Thus, although a primary role of early tumour suppressor genes might be related to wound repair and regeneration rather than control of tumours [7] , one might expect to find tumours in all animals, including the most simple ones. 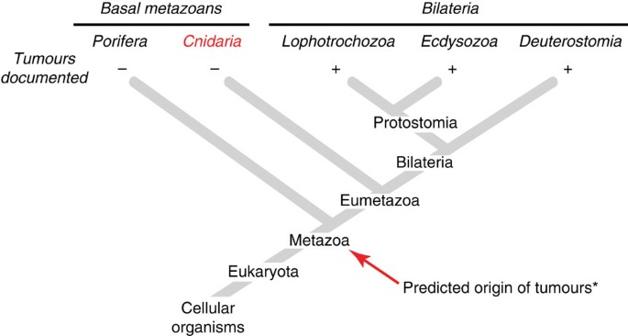Figure 1: Spontaneously occurring tumours are not reported in animals outside the bilaterian clade. Schematic phylogenetic tree showing main branches of metazoan evolution and position of Cnidaria inside the group of pre-bilaterian metazoans. The clades where cases of spontaneously occurringbona fidetumours have been documented are marked by + sign. Phylostratigraphic analysis of genes associated with cancer in humans indicates their early evolutionary emergence and predicts the evolutionary origin of animal tumours to lie in the root of metazoan tree6. This does not preclude the possibility that tumour suppressor-related genes in early metazoan evolution were involved in the control of cell proliferation to adjust to environmental changes7. Figure 1: Spontaneously occurring tumours are not reported in animals outside the bilaterian clade. Schematic phylogenetic tree showing main branches of metazoan evolution and position of Cnidaria inside the group of pre-bilaterian metazoans. The clades where cases of spontaneously occurring bona fide tumours have been documented are marked by + sign. Phylostratigraphic analysis of genes associated with cancer in humans indicates their early evolutionary emergence and predicts the evolutionary origin of animal tumours to lie in the root of metazoan tree [6] . This does not preclude the possibility that tumour suppressor-related genes in early metazoan evolution were involved in the control of cell proliferation to adjust to environmental changes [7] . Full size image Hydra , a freshwater polyp belonging to the cnidarian clade [8] , [9] , has a very simple body plan composed of only two cell layers, which are maintained by three independent stem cell lineages [10] . Besides the two epithelial stem cell lineages, polyps possess multipotent interstitial stem cells (ISCs), which are capable to differentiate to a number of somatic cell types and to germline cells [10] , [11] , [12] . Gametogenesis in Hydra , which is triggered by changes in environmental conditions [13] , [14] , involves mitotic proliferation of committed precursor cells followed by terminal differentiation into eggs and sperm. Despite the apparent morphological simplicity of the Hydra body plan, the proliferation and differentiation behaviour of the cell lineages is tightly controlled [15] , [16] , allowing stable maintenance of tissue homeostasis for extended periods. In fact, due to the asexual mode of reproduction by budding Hydra is one of the very few examples of animals, which appear to be effectively immortal [17] , [18] . Here we provide evidence that differentiation of ISCs into female gametes can be disturbed resulting in spontaneously occurring transplantable tumours in two species of Hydra . Morphology and histology Initially, we observed a single polyp in each of two species, Hydra oligactis and Pelmatohydra robusta , which showed severely altered morphology never seen before in long-term mass cultures ( Fig. 2a ). These individuals carrying morphologically similar tumour-like abnormalities served to establish clonal lines in each species, which have been successfully kept in the lab for more than 5 years (see Methods). 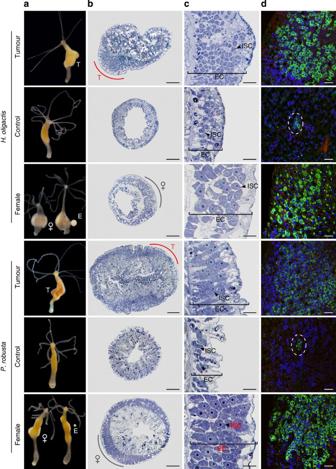Figure 2: The tumour in two species ofHydrais formed by accumulation of ISCs. (a) Morphology of tumorous (tumour), normal (control) and oogenesis-induced (female) polyps ofH. oligactisandP. robusta. Abnormal tumorous tissue (T), developing female gonad at oogenesis stage 3–4 (♀) and mature egg (E) are indicated. (b) Cross-sections through polyp body column demonstrate swelling of the ectodermal tissue in tumorous polyps (T), resembling female gonad (♀) at early oogenesis stages (1–3). InH. oligactis, tumour tends to be localized to one side of the body column, whereas inP. robustamultiple local accumulations of interstitial-like cells can be seen on histological sections. Scale bar, 50 μm. (c) ISC are accumulated in the ectodermal tissue layer (EC) in tumorous polyps and in females undergoing oogenesis. Scale bar, 15 μm. (d) Immunostaining reveals abundant cells positive for germline marker periculin inside the tumour tissue and female gonads. In control polyps only rare periculin-positive germline cells are observed (outlined). Scale bar, 50 μm. Figure 2: The tumour in two species of Hydra is formed by accumulation of ISCs. ( a ) Morphology of tumorous (tumour), normal (control) and oogenesis-induced (female) polyps of H. oligactis and P. robusta . Abnormal tumorous tissue (T), developing female gonad at oogenesis stage 3–4 (♀) and mature egg (E) are indicated. ( b ) Cross-sections through polyp body column demonstrate swelling of the ectodermal tissue in tumorous polyps (T), resembling female gonad (♀) at early oogenesis stages (1–3). In H. oligactis , tumour tends to be localized to one side of the body column, whereas in P. robusta multiple local accumulations of interstitial-like cells can be seen on histological sections. Scale bar, 50 μm. ( c ) ISC are accumulated in the ectodermal tissue layer (EC) in tumorous polyps and in females undergoing oogenesis. Scale bar, 15 μm. ( d ) Immunostaining reveals abundant cells positive for germline marker periculin inside the tumour tissue and female gonads. In control polyps only rare periculin-positive germline cells are observed (outlined). Scale bar, 50 μm. Full size image To get first insight into the cellular nature of the observed alterations, we subjected animals of both lines to a histological analysis. Figure 2b,c shows that the abnormal tissue bulges contain increased numbers of cells with interstitial cell morphology, accumulated within the ectodermal epithelial layer. These interstitial cells are clustered, contain large nuclei with 1–2 dense nucleoli and undifferentiated granulated cytoplasm ( Fig. 2c and Supplementary Figs 1 and 2 ), and do not show any specific features characteristic for somatic derivatives of ISCs—nematocytes, neurons or gland cells [19] . Conversely, the tumour cells resemble in size and morphology large germ cells, described as ‘germ cell II’ (GCII) [20] , which can be observed in early stages of oogenesis (stage 1–3 (ref. 21 ), Supplementary Figs 1a–d and 2 ). In normal polyps, GCII cells appear in the ectoderm of female polyps only after oogenesis is initiated by environmental stimulus. Within 96 h they differentiate into GCIII and GCIV cells ( Supplementary Figs 1a,c and 2 ), and finally give rise to a single oocyte and numerous nurse cells, which are phagocytized by an oocyte [20] . In tumorous polyps, GCII-like cells are permanently present, their differentiation is not dependent on environmental stimuli and they were never observed to further differentiate into oocytes or nurse cells ( Fig. 2b,c and Supplementary Figs 1 and 2 ). In contrast to females, the endoderm in tumour polyps is also morphologically altered. The overall changes in morphology, the appearance of these tumour-like structures and the cellular characteristics were found to be similar in both species ( Fig. 2 and Supplementary Fig. 1 ). Detection of female-specific markers To characterize the cell type involved in tumorigenesis in more detail, we employed molecular markers specific for Hydra ’s germ-line restricted ISCs. In situ hybridization with a Cnnos1 -specific probe [16] , [22] revealed in both lines that tumours are composed, at least in part, of interstitial cells expressing the Cnnos1 gene ( Supplementary Fig. 3 ). Immunocytochemistry with an antibody against periculin protein, known to label Hydra ’s female germline precursor cells [23] , revealed that in both lines the interstitial cells in the tumour tissue are expressing this female-specific marker ( Fig. 2d and Supplementary Fig. 1e–h ). Although periculin expression is activated not only during oogenesis but also by a number of environmental signals [23] , the observation of tumour cells expressing both Cnnos1 and periculin supports the view that tumour cells are committed to the female germline. A quantitative morphological analysis showed that the cells within tumours are predominantly large ISCs [19] ( Fig. 3a ). The increase in the proportion of large ISCs is a characteristic feature of early (stage 1–3) phase of oogenesis [20] . 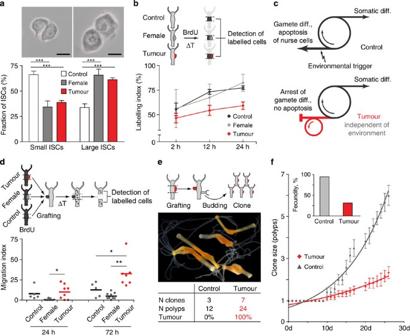Figure 3: Cellular behaviour of the tumour and its fitness consequences inP. robustaline. (a) Large ISCs19(inset, phase-contrast microscopy) represent dominant fraction of interstitial cells in tumour tissue and in female gonads. This contrasts the control tissue (n=8 control,n=6 female,n=13 tumour; scale bar, 10 μm). (b) BrdU labelling (experiment outline, top) reveals that there is no increase in proliferation of interstitial cells in tumour tissue compared with control and oogenesis-induced polyps. Only ~\n60% of tumour cells enter cell cycle within 24 h of labelling (n=5 control,n=5 female,n=5 tumour at each time point). (c) A model of theHydratumour growth. In healthy polyps (control), ISCs cycle and produce cells of somatic differentiation. They enter gamete differentiation only in the presence of environmental trigger, and give rise to a single oocyte and numerous nurse cells, which undergo apoptosis. In tumour tissue, ISCs become committed to germline differentiation independently of environment, their maturation is arrested and the cells are not eliminated by apoptosis. (d) Transplantation and tracing of BrdU-labelled cells (experiment outline, top) reveal tumour cells to migrate into normal host tissue at increased rates compared with control and female gonad cells (24 h post transplantation:n=5 control,n=7 female,n=8 tumour; 72 h post transplantation:n=5 control,n=9 female,n=7 tumour). (e) Tumour grafts transplanted into healthy hosts (experiment outline, top) induce new tumours in the recipient polyps and in their clonal progeny. All clonal progeny (n=24) derived from seven recipient clonal lines demonstrate tumorous phenotype. (f) Growth curves for tumour and controlP. robustacultures demonstrate tumour impact on population growth rate; exponential fit curves,n=12 for each line; doubling time 8.1 days (95% confidential interval, 7.6–8.7) for control, 18.2 days (15.8–21.4) for tumour line. Capability to produce eggs (fecundity, inset) is reduced in tumorous polyps (n=41) in comparison with control (n=39). Tumorous polyps are 2.99 times less likely to develop eggs, than normal polyps, with odds ratio 39.85, Fisher’s exact test two-tailedP=1.7E−9. Error bars in all panels represent±one s.e.m., (*P<0.05; **P<0.01, ***P<0.001; one-way analysis of variance with Bonferronipost hoctest). Figure 3: Cellular behaviour of the tumour and its fitness consequences in P. robusta line. ( a ) Large ISCs [19] (inset, phase-contrast microscopy) represent dominant fraction of interstitial cells in tumour tissue and in female gonads. This contrasts the control tissue ( n= 8 control, n= 6 female, n= 13 tumour; scale bar, 10 μm). ( b ) BrdU labelling (experiment outline, top) reveals that there is no increase in proliferation of interstitial cells in tumour tissue compared with control and oogenesis-induced polyps. Only ~\n60% of tumour cells enter cell cycle within 24 h of labelling ( n= 5 control, n =5 female, n =5 tumour at each time point). ( c ) A model of the Hydra tumour growth. In healthy polyps (control), ISCs cycle and produce cells of somatic differentiation. They enter gamete differentiation only in the presence of environmental trigger, and give rise to a single oocyte and numerous nurse cells, which undergo apoptosis. In tumour tissue, ISCs become committed to germline differentiation independently of environment, their maturation is arrested and the cells are not eliminated by apoptosis. ( d ) Transplantation and tracing of BrdU-labelled cells (experiment outline, top) reveal tumour cells to migrate into normal host tissue at increased rates compared with control and female gonad cells (24 h post transplantation: n= 5 control, n= 7 female, n= 8 tumour; 72 h post transplantation: n= 5 control, n= 9 female, n= 7 tumour). ( e ) Tumour grafts transplanted into healthy hosts (experiment outline, top) induce new tumours in the recipient polyps and in their clonal progeny. All clonal progeny ( n =24) derived from seven recipient clonal lines demonstrate tumorous phenotype. ( f ) Growth curves for tumour and control P. robusta cultures demonstrate tumour impact on population growth rate; exponential fit curves, n =12 for each line; doubling time 8.1 days (95% confidential interval, 7.6–8.7) for control, 18.2 days (15.8–21.4) for tumour line. Capability to produce eggs (fecundity, inset) is reduced in tumorous polyps ( n =41) in comparison with control ( n =39). Tumorous polyps are 2.99 times less likely to develop eggs, than normal polyps, with odds ratio 39.85, Fisher’s exact test two-tailed P =1.7E−9. Error bars in all panels represent±one s.e.m., (* P <0.05; ** P <0.01, *** P <0.001; one-way analysis of variance with Bonferroni post hoc test). Full size image Cell proliferation analysis Tumours in vertebrates may develop either due to increased proliferation rate or due to arrest of terminal differentiation (for example, in teratocarcinomas) [24] , [25] . To examine the proliferation capacity of the tumour cells, we performed continuous bromodeoxyuridine (BrdU) labelling experiment in the Pelmatohydra robusta line. In this and similar experiments shown below, we used only P. robusta , as very slow propagation of tumour-bearing polyps precluded any extensive experimentation in H. oligactis (see Methods). Continuous labelling revealed that although interstitial cells from control polyps show the well-described labelling dynamics [26] with ~\n80% cells labelled after 24 h ( Fig. 3b ), the proportion of labelled cells from tumour tissue is only ~\n60%, indicating that in tumours lower fraction of cells have entered cell cycle. These observations clearly indicate that the increase of cells in tumours is not caused by increased proliferative activity of ISCs. Apoptosis analysis As apoptosis of nurse cells is an essential step of normal oogenesis [27] , we next examined apoptotic activity in tumorous polyps. Analysis by terminal deoxynucleotidyl transferase dUTP nick-end labelling (TUNEL) assay ( Supplementary Fig. 4 ) and acridine orange staining ( Supplementary Fig. 5 ) revealed no increase in apoptosis activity in H. oligactis tumorous polyps compared with that in normal asexual animals, while egg patches in females showed the previously observed [27] massive apoptosis. This suggests that tumour cells might be resistant to apoptotic control mechanisms. Transplantation assay In both Hydra species, daughter polyps originating by budding of the tumorous polyps were typically observed to bear tumours as well, indicating that tumour cells might be able to spread in unaffected host tissue and induce new tumours. To examine the disseminating potential of Hydra tumour cells, we performed transplantation experiments, where we followed migration of the BrdU-labelled tumour cells into the host tissue outside the transplantation region. Figure 3d shows that cells from the tumour donor tissue invade normal host tissue at increased rates compared with controls. Labelled cells transplanted into the middle of the host body can be detected even at the oral and aboral ends of the body column, indicating that these cells are able to migrate over large distances ( Fig. 3d ). This migratory activity appears to resemble cell behaviour in invasive mammalian tumours [1] . Moreover, tumour grafts transplanted into healthy hosts were capable to induce new tumours in both the recipient adult polyps as well as in their clonal progeny ( Fig. 3e ). These observations point to an environment-independent and, therefore, autonomous growth of Hydra tumour cells. Assessment of fitness One of the inherent properties of malignant tumours is that diseased individuals have reduced fitness. To estimate how tumours influence the fitness of Hydra , we compared the growth rate and fecundity of P. robusta tumorous and control polyps. Figure 3f shows that tumour-bearing polyps have a drastically reduced population growth rate with a twofold increased population doubling time. In addition, tumour-bearing polyps have a significantly reduced capacity of egg production ( Fig. 3f ). Thus, asexual propagation by budding as well as sexual reproduction is strongly affected in tumour-bearing polyps. The reduced fitness components indicate that the observed tissue abnormalities compromise the health of the P. robusta animals and therefore act as a disease. Although we were not able to directly measure fitness components of H. oligactis tumour-bearing polyps, the extremely slow propagation in culture and almost negligible egg production of this line suggests that its fitness is even more affected compared with that of P. robusta . Transcriptome analysis To get unbiased insight into the gene expression profiles in tumours compared with controls, we next sequenced the transcriptome of H. oligactis and performed microarray experiments. The severity of tumour phenotype in H. oligactis prioritized this species for the transcriptome analysis. Sequencing of transcripts from pooled asexual adults, buds, females at various phases (stage 1–7) of oogenesis and tumour polyps resulted in 690,540 reads (~\n224 Mb) that we assembled after filtering into 31,473 contigs (~\n20 Mb) that ranged from 100 to 11,823 bp in size, with an average contig length of 662 bp and N50 of 852 bp. These contigs served as a template for designing an H. oligactis Agilent microarray, which was subsequently hybridized to cRNAs from tumour, female and asexual animals. For further analysis we only used contigs that contained well-supported open reading frames (22,719 in total). To reveal the global changes in gene expression associated with tumour formation in Hydra , we analysed the results of microarray hybridization by principle component analysis ( Fig. 4a ). The first two principle component vectors together explain 76.3% of the expression variance and clearly separate the H. oligactis tumour transcriptome from the transcriptomes of both asexual controls and females ( Fig. 4a ). 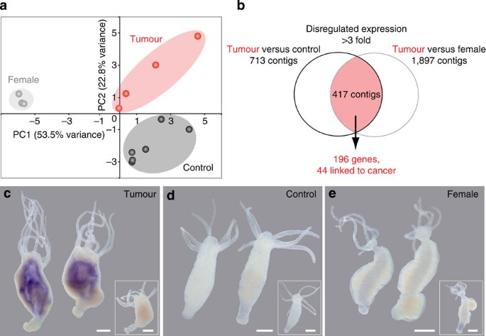Figure 4:H. oligactistumour-bearing polyps have a unique gene expression profile. (a) Principal component analysis separates transcriptomes of tumour, oogenesis-induced (female) and controlH. oligactispolyps. Percentage of explained variance is indicated for each component. (b) Venn diagram representing differentially regulated (>3.0-fold change) contigs in tumour polyps compared with control and female polyps. The overlap between both groups contains 417 contigs and makes a specific signature of the tumour transcriptome. Among these contigs, 196 uniquely correspond toH. magnipapillatagene models, and 44 of them show homology to genes implicated in mammalian malignancies. (c–e) Whole-mountin situhybridization with DIG-labelled antisense RNA probe specific forHydrahomologue oftranslationally controlledtumour-protein(tpt1, p23) gene confirms, thattpt1is expressed exclusively in tumorous polyps (tumour,c), with no specific signal being detected in normal asexual (control,d) or oogenesis-induced (female,e) polyps. Hybridization with sense-probe (insets) reveals no signal, confirming detection specificity. Scale bar, 300 μm. Figure 4a also shows that the overall expression divergence between female and control transcriptomes is larger than the expression divergence between tumours and asexual controls, indicating that the molecular signature of tumour cells differs greatly from that in females. Quantitative PCR analysis confirmed ( Supplementary Fig. 6 ) that tumours have very distinct gene expression profile, different from female gonads at either early or late stages of oogenesis. Taken together, although several molecular markers are shared (periculin, Cnnos1 — Fig. 2d and Supplementary Figs 1 and 3 ), the overall gene expression profile in H. oligactis tumours is clearly different from that in females undergoing oogenesis. Figure 4: H. oligactis tumour-bearing polyps have a unique gene expression profile. ( a ) Principal component analysis separates transcriptomes of tumour, oogenesis-induced (female) and control H. oligactis polyps. Percentage of explained variance is indicated for each component. ( b ) Venn diagram representing differentially regulated (>3.0-fold change) contigs in tumour polyps compared with control and female polyps. The overlap between both groups contains 417 contigs and makes a specific signature of the tumour transcriptome. Among these contigs, 196 uniquely correspond to H. magnipapillata gene models, and 44 of them show homology to genes implicated in mammalian malignancies. ( c – e ) Whole-mount in situ hybridization with DIG-labelled antisense RNA probe specific for Hydra homologue of translationally controlled tumour -protein ( tpt1, p23 ) gene confirms, that tpt1 is expressed exclusively in tumorous polyps (tumour, c ), with no specific signal being detected in normal asexual (control, d ) or oogenesis-induced (female, e ) polyps. Hybridization with sense-probe (insets) reveals no signal, confirming detection specificity. Scale bar, 300 μm. Full size image To recover the specific signature in the transcriptome of H. oligactis tumours, we identified contigs that show high, consistent and significant deregulation of expression compared with females and asexual controls ( Fig. 4b ). From the pool of 417 contigs that showed more than threefold difference, we extracted a non-redundant set of 196 contigs that reliably correspond to the Hydra magnipapillata gene models [28] ( Supplementary Data 1 ). Out of these 196 contigs, we found 44 to represent Hydra genes with homology to genes implicated in mammalian tumours (Fig. 4b and Supplementary Data 1 ). Predicted functional properties of these genes encompass many functions that are thought to be hallmarks of cancer in mammals [1] , [29] . Examples include genes affecting cell cycle, apoptosis, genomic stability and metabolism ( Supplementary Data 1 ). It is also indicative that the tumour-specific transcriptome contains numerous non-conserved ‘taxonomically restricted genes’ as well as a number of conserved genes, not yet found to be associated with tumour cells in vertebrates ( Supplementary Data 1 ). Slow propagation of tumour cultures precluded any large-scale screen of tumour-specific genes for expression profiles by in situ hybridizations. However, by real-time PCR analysis ( Supplementary Data 2 ) we validated the transcriptome analysis and explicitly assessed the expression levels of genes potentially connected with the hallmarks of cancer. By analysing 27 tumour-specific and control genes ( Supplementary Data 2 ) we were able to prioritize for in situ expression analysis a Hydra gene homologous to human tpt1 gene (translationally controlled tumour protein, p23 ), which is implicated in many mammalian tumours and is known to have anti-apoptotic activity [30] . This gene showed drastic upregulation in the tumorous Hydra polyps ( Fig. 4c , Supplementary Data 2 and Supplementary Fig. 6 ). In sharp contrast, in female ( Fig. 4e ) and asexual control polyps ( Fig. 4d ) expression of this gene could not be detected by in situ hybridization. These gene expression data are in full agreement with the observation ( Supplementary Figs 4 and 5 ) of low apoptosis activity in tumorous polyps. With regard to the observation ( Fig. 3d ) that Hydra tumour cells display disseminating behaviour, it was interesting to note that Hydra genes encoding matrix metalloproteinase proteins in the large majority of cases are not upregulated in tumours ( Supplementary Data 3 ). This leaves open the question on the precise role of matrix metalloproteinases in the observed disseminating behaviour of tumour cells in Hydra . Another potentially interesting question not yet answered relates to how Hydra ’s tumour cells evolved the properties enabling them to survive and proliferate despite the mechanisms that have emerged to constrain them. The advent of next-generation sequencing technologies now seems to offer a unique opportunity in understanding the genomic forces that govern tumour initiation in a multicellular organism at the base of animal evolution. Taken together, our observations reveal that Hydra tumours are composed of interstitial cells morphologically similar to female germline precursor cells ( Fig. 2 and Supplementary Figs 1 and 2 ). Our findings also indicate that tumour cells express molecular markers characteristic to Hydra ’s female-restricted interstitial cell lineage ( Fig. 2 and Supplementary Figs 1 and 3 ). In contrast to normal female precursor cells, tumour cells appear not to be able to terminally differentiate into oocytes and nurse cells ( Supplementary Figs 1 and 2 ), do not show increase in proliferation activity ( Fig. 3b ) and are not removed by apoptosis ( Supplementary Figs 4 and 5 ). Hydra tumour cells also acquire a new phenotype that is reflected in their autonomous growth, insensitivity to environmental stimuli and increased migratory potential ( Fig. 3 and Supplementary Figs 3 and 7 ). Under this scenario, a plausible mechanistic reason for the uncontrolled accumulation of interstitial cells in Hydra tumours is differentiation arrest of committed female precursor cells ( Fig. 3c and Supplementary Fig. 7 ). As, however, global expression patterns show ( Fig. 4 and Supplementary Fig. 6 ) that Hydra tumour cells have a specific expression profile differing from that of normal female germline cells, the exact origin of the Hydra tumour cells still remains to be resolved. Another uncertainty in determining the precise cellular origin of the tumour cells relates to the anti-periculin1a antibody that we used for the immunostaining studies. This polyclonal antibody that was raised against periculin1a in Hydra vulgaris recognizes multiple paralogues of periculin [23] . This property of the anti-periculin antibody, the presence of at least four periculin paralogues in H. oligactis and possible expression of some of the periculin paralogues outside the context of female germline preclude any firm conclusion about cellular origin of the tumour cells. We therefore consider our model of tumour formation through differentiation arrest of committed female precursor ( Supplementary Fig. 7 ) still tentative and expect that unambiguous markers together with functional evidences will resolve this issue in the future. In conclusion, our study indicates that naturally occurring tumour formation can be observed in pre-bilaterian cnidarians. Cellular and molecular properties of Hydra ’s tumour cells appear to demonstrate some parallels with the previously described hallmarks of cancer cells in vertebrates [1] . Therefore, it appears that spontaneous tumours are plesiomorphic characters of Bilateria and are not derived features of distinct bilaterian lineages. As Hydra is a rare example of an animal that can control senescence, our findings also imply that even a literally immortal organism is not immune from developing disseminating and fitness reducing tumours. Animals and culture conditions Experiments were carried out using H. oligactis strain St. Petersburg and P. robusta strain L7. Animals of both strains were used for histological and immunohistochemical examinations and in situ hybridization experiments. Owing to the poor viability of tumour-bearing polyps and slow clonal propagation rate of H. oligactis tumour culture, we used only P. robusta tumour-bearing polyps for cell proliferation, migration and fitness assays. Conversely, the severity of the tumour phenotype in H. oligactis prioritized this strain for transcriptome sequencing and microarray analysis. Animals of all strains were maintained under constant environmental conditions, including culture medium, food and temperature (18 °C) according to standard procedures [31] . Oogenesis was induced by lowering the culture temperature to 10 °C and depriving animals of food [13] for a period of 14 ( H. oligactis ) or 30 days ( P. robusta) . Single tumour-bearing polyps, which we discovered by careful observations, appeared spontaneously and independently in the mass cultures of both species. These founder polyps were asexually propagated by budding or by cutting longitudinally in two halves to establish clonal cultures, which have been maintained in the lab for more than 5 years. Tumour grows progressively with time, but typically does not kill the host. Affected polyps are able to feed and also to bud, thus still showing asexual mode of reproduction. In the case of P. robusta , the daughter polyp originated by budding of parental tumorous polyp is tumorous in 100% cases. Offspring develops tumour in normal laboratory conditions, without any stimulation and condition changes. In H. oligactis , very rarely apparently healthy polyps detach from the tumorous parental polyps. If these polyps did not develop any visible tumour in 1–2 months, we removed them from the culture and excluded them from further analysis. Histological staining For histological analysis, polyps were relaxed in 2% urethane and fixed with 4% formaldehyde, dehydrated in ethanol and embedded into LR-White resin (Ted Pella, Redding, CA, USA) according to the manufacturer’s instruction. Semi-thin sections (0.5 μm thick) were cut using Ultracut S ultratome, mounted on slides and stained with methylene blue/azur II as described previously [32] , [33] . Light microscopy images were taken on a Zeiss Axioscope microscope equipped with Axiocam digital camera (Zeiss, Jena, Germany). Immunohistochemistry Immunohistochemical detection of periculin protein in whole mount Hydra preparations was performed as described previously [23] using polyclonal mouse antisera against periculin1a protein (1:500 diluted, produced by T. Bosch lab) and Alexa488-conjugated donkey-anti-mouse secondary antibodies (2 μg ml −1 ; Invitrogen, Eugene, OR, USA). Rhodamin-phalloidin and TO-PRO3 counterstaining was conducted as described previously [34] . Confocal laser-scanning microscopy was done using a TCS SP1 laser-scanning confocal microscope (Leica, Wetzlar, Germany). In situ hybridization Expression patterns of Cnnos1 and tpt1 genes were detected in whole mount Hydra preparation by in situ hybridization with digoxigenin (DIG)-labelled RNA probes [32] . Anti-sense RNA probes were designed to recognize specifically the sequence of Hydra Cnnos1 gene product (GenBank XM_002161814.1) and transcript of H. oligactis (contig 19403) homologous to human tpt1 gene ( tpt1 , p23 , GenBank XM_002157314.2 in H. magnipapillata ). DIG-labelled sense probes were used as a control. Signal was developed using anti-DIG antibodies conjugated to alkaline phosphatase (1:2000, Roche Diagnostics, Mannheim, Germany) and NBT/BCIP staining solution (Roche). Images of in situ preparations were collected on a Zeiss Axioscope microscope with Axiocam camera. Cell-type and proliferation assays Tissue maceration technique [19] was used to analyse the cell composition of tumorous, normal and female gonad tissue in H. oligactis and P. robusta . Middle body-column region, containing tumorous tissue, developing female gonad (egg patch at stages 1–5 of oogenesis [20] ) or normal tissue, was excised, macerated into single-cell suspension, fixed with 8% formaldehyde and dried on slides as described previously [19] . For quantitative morphological analysis we used in total 8 control P. robusta polyps, 6 female and 13 tumorous polyps. On examination of the slides using phase-contrast and differential interference contrast microscopy, we counted large and small ISCs [19] separately. In this and similar experiments, a blind-control design was implemented, so that the investigator was unaware of the sample group allocation when assessing the experiment outcome. In total 7,952 cells were counted on slides (611.7±33.1; mean±s.e.m. cells per slide; n =13) made from macerated tumour tissue, 3,795 cells on slides (474.4±43.3; n =8) from control tissue and 3,161 cells on slides (526.8±24.9; n =6) made from female gonad tissue. P. robusta polyps were used for cell proliferation activity assessment using BrdU-labelling technique. Polyps were incubated in 5 mmol l −1 BrdU (Sigma, Steinheim, Germany) solution for 2–24 h (continuous labelling), with the solution being additionally injected into the polyp gastric cavity every 6 h. After 2, 12 or 24 h of incubation, the middle body-column region, containing tumorous tissue, developing female gonad (egg-patch) or normal tissue was excised and macerated into single-cell suspension [19] . In total we used five polyps of each sort for every time point (2, 12 and 24 h) of continuous labelling experiment. Immunodetection of BrdU on slides was done as described previously [15] using monoclonal anti-BrdU antibodies (1:100, Roche), alkaline phosphatase-conjugated sheep-anti-mouse secondary antibodies (1:5,000, Millipore, Melbourne, Australia) and NBT/BCIP staining solution (Roche). In continuous labelling experiment, BrdU-labelling index was assessed for all interstitial cells together, without discriminating large and small ISCs. For all samples (tumour, control, female) at each time point (2, 12 and 24 h) we prepared five slides. In average we counted 990.3±39.1 (2 h; n =5), 825.0±28.8 (12 h; n =5) and 1,062.8±88.8 (24 h; n =5) cells on slides made from macerated tumour tissue; 827.0±63.7 (2 h; n =5), 638.8±36.4 (12 h; n =5) and 1,006.2±88.0 (24 h; n =5) cells on slides made from macerated control tissue; and 906.3±34.5 (2 h; n =5), 768.5±65.5 (12 h; n =5) and 877.3±36.4 (24 h; n =5) cells on slides made from macerated female gonad tissue. Statistical analysis of the data was carried out using one-way analysis of variance with Bonferroni post hoc test. Cell migration assays Migratory activity of the interstitial cells was examined in P. robusta strain. Donor polyps were labelled with BrdU for 24 h, and a 4–6 mm 3 piece of tumour tissue, normal control tissue or developing female gonad (oogenesis stage 2–3) was laterally grafted into the middle body part of healthy unlabelled polyp according to the transplantation procedure described by Takano and Sugiyama [35] . We excised, pooled and macerated oral and aboral part of the recipient body column at 24 and 72 h after transplantation. Immunodetection of BrdU on slides was done as described above. On examination of the slides using phase-contrast microscopy, we counted BrdU-positive ISCs and non-labelled epithelial cells. To calculate migration index, we normalized the number of BrdU-positive ISCs by the number of non-labelled epithelial cells. To control for the occasional contamination of the recipient tissue with the donor epithelial tissue, we discarded from the analysis the slides that showed >1% of the BrdU-positive epithelial cells. In total, 20 grafts were analysed at 24 h (controls: n =5; female gonads: n =7; tumours: n =8) and 21 grafts at 72 h after transplantation (controls: n =5; female gonads: n =9; tumours: n =7). In total 17,731 cells were counted (432.5±7.2 cells per slide). The data were analysed using one-way analysis of variance with Bonferroni post hoc test. To check whether the tumorous cells invading normal host tissue are able to induce de novo tumour formation, we grafted small pieces of unlabelled tumour tissue into the healthy hosts. We fed the host polyps ad libitum daily, and 35 days after transplantation we screened the clonal progeny generated by the budding for the presence of tumours. In total, we analysed seven clonal lines with grafted tumours and three control lines, where healthy tissue was transplanted. Apoptosis analysis Apoptosis activity in H. oligactis tumour-bearing, control polyps and female polyps at different oogenesis phases (stage 1–7) was analysed by TUNEL assay and acridine orange staining as described previously [27] . In TUNEL experiment, polyps were relaxed in 2% urethane, fixed with 4% formaldehyde and treated with 150 U ml -1 TdT enzyme (Fermentas) in the presence of 5 μmol l −1 DIG-dUTP for 2 h at 37 °C. Detection of incorporated DIG was performed as in in situ hybridization experiments. To detect apoptotic cells in vivo , polyps were stained 10 min in 1 μg ml −1 acridine orange (Sigma) solution, relaxed in 2% urethane and monitored under Zeiss Axioscope microscope with Axiocam camera and fluorescein isothiocyanate filter set. Confocal laser-scanning microscopy was done using a TCS SP1 laser scanning confocal microscope (Leica, Wetzlar, Germany). Fitness assays To assess the growth rate we established P. robusta clonal lines of tumour-bearing ( n =12) and normal polyps ( n =12) by putting one founder polyp per well into a 24-well plate. The polyps were fed daily ad libitum. The number of clonal progeny propagated by budding within each clonal line was counted daily for a period of 4 weeks. To estimate fecundity, tumour-bearing ( n =41) and normal ( n =39) polyps were kept at 10 °C and deprived of food for 30 days. After this period we counted the number of tumour-bearing and normal polyps that produced eggs. These data were used to generate four-field contingency table and to calculate further odds ratio value for egg production by tumorous polyps compared with control polyps. The statistical significance of fecundity was analysed by Fisher’s exact test. Transcriptome sequencing and assembly For transcriptome sequencing, mRNA was isolated from a pool of normal, tumorous and oogenesis-induced (stage 1–7 (ref. 20 )) H. oligactis polyps using Illustra QuickPrep Micro mRNA purification kit (GE Healthcare, Buckinghamshire, UK). A double-stranded complementary DNA library was constructed using SMARTer PCR cDNA Synthesis Kit (Clontech Laboratories, Mountain View, CA, USA). The cDNA library, representing the complete transcriptome of H. oligactis , was pyrosequenced on Roche FLX 454 sequencer as explained elsewhere [16] . After removal of adaptor sequences, 690,540 reads (~\n224 Mb) were assembled into contigs using the Newbler 2.5.5 assembly pipeline. After filtering, this yielded 31,473 contigs (~\n20 Mb) of 100–11,823 bp in size, with an average contig length of 662 bp and N50 of 852 bp. Microarray hybridization and analysis Custom Agilent Gene Expression Microarray was designed using the H. oligactis transcriptome (31,473 contigs, 4 × 44 k platform). For the microarray analysis of gene expression, total RNA was isolated from H. oligactis healthy control ( n =6 replicates), tumour-bearing polyps ( n =4) and oogenesis-induced polyps (pooled equal ratios of stages 1–7 (ref. 20 ) of oogenesis, n =3) by TRIzol reagent (Invitrogen) according to the manufacturer’s instructions. After chloroform extraction, the aqueous phase was purified on the RNA-binding cartridge of PureLink RNA Mini Kit (Ambion, Life Technologies, Darmstadt, Germany) according to the protocol of the manufacturer. The RNA samples were additionally purified by glycogen–potassium acetate precipitation followed by washing with ice-cold 80% ethanol. About 400 ng of total RNA were labelled with Cy3 using the one-colour Quick-Amp Labeling Kit (Agilent Technologies, Waldbronn, Germany). Labelled cRNA samples ( n =13 in total) were hybridized to custom Agilent Gene Expression Microarray 4 × 44 k slides for 17 h at 65 °C and treated according to the Agilent protocol. The microarrays were scanned using the Agilent High Resolution G2565CA Microarray Scanner System. Raw microarray image files were processed and quality checked by Agilent Feature Extraction 10.7.3 software. The microarray and custom-design data were deposited at the NCBI Gene Expression Omnibus repository under the accession number GSE56287. Background-subtracted signal intensity values that contain correction for multiplicative surface trends (gProcessedSignal) generated by Feature Extraction Software were used for further data analysis. Using GeneSpring microarray data analysis software, we filtered probes that were flagged as non-uniform or as population outliers. We additionally filtered data set for expression levels of contigs that lack evidence to code for proteins. The potential coding regions were initially predicted by ESTscan [36] and then double checked by BLASTp analysis against H. magnipapillata gene predictions [28] . This procedure reduced the expression sample to 22,719 contigs that were used in the subsequent analyses. This data set was normalized by 75th percentile normalization procedure as recommended by Agilent. To reveal the global changes in gene expression patterns, we performed principal component analysis using NIPALS algorithm. To assess the putative functional properties of the contigs that most probably code for proteins, we performed sequence similarity searches against the NCBI nr database and the predicted human genes. Significance of differences in the pairwise comparisons between tumours and controls were conducted by Student’s t -test with false discovery rate correction. By setting a threshold of >3.0-fold change in relation to healthy control and oogenesis-induced females, we obtained a set of 417 significantly differentially regulated contigs ( P ≤0.05). This set was further reduced by keeping only contigs that had the most significant e -value in the situations where several contigs from the full data set (22,719 contigs) had the same H. magnipapillata gene as the best BLAST match. This procedure yielded 196 contigs that were significantly differentially expressed above the threshold of 3.0-fold change and have the best correspondence to the H. magnipapillata gene models. Finally, by manual screen of the literature and sequence databases, we were able to link 44 of these genes to mammalian homologues that are implicated in tumours. Quantitative real-time PCR gene expression analysis To validate the results of microarray hybridization analysis and to find most promising genes for expression analysis by in situ hybridization, we performed quantitative real-time PCR. We used the same total RNA samples that we isolated in microarray experiment: RNA from H. oligactis healthy controls ( n =2), tumour-bearing polyps ( n =2) and oogenesis-induced polyps ( n =2). cDNA samples were produced using First Strand cDNA Synthesis Kit (Thermo Scientific, Schwerte, Germany). Real-time PCR was performed using GoTaq qPCR Master Mix (Promega, Madison, USA) and oligonucleotide primers specifically designed to recognize H. oligactis genes ( Supplementary Table 1 ). In total, we assessed expression level of 27 genes, including house-keeping genes, oogenesis-related and tumour-specific genes. The data were collected by ABI 7300 Real-Time PCR System (Applied Biosystems, Foster City, USA) and analysed by conventional ddCt method, using expression level of EF1a ( translation elongation factor 1 alpha) gene as equilibration reference. The experiments were repeated twice, resulting in two biological with two technical replicates each. These data were used further to calculate mean fold change factors of gene expression in tumour related to healthy asexual polyps (Tumour versus Control, Supplementary Data 2 ) or related to oogenesis-induced animals (Tumour versus Female, Supplementary Data 2 ). To compare expression level of 27 genes in H. oligactis tumorous tissue with female gonad tissue at different oogenesis stages, we excised tumorous tissue ( n =10), developing female gonads at early (stage 1–3; n =10), and late (stage 4–7; n =10) oogenesis and normal tissue ( n =10) from 10 polyps of each type. These samples were further used for RNA extraction, cDNA synthesis and PCR amplification as described above. The experiments were repeated twice, resulting in two biological replicates with two technical replicates each. These data were used further to calculate mean fold change factors of gene expression in tumorous tissue, early and late female gonad related to healthy asexual tissue ( Supplementary Fig. 6 ). Accession codes: Raw transcriptome sequencing data have been deposited in the Sequence Read Archive at the National Center for Biotechnology Information (NCBI) under accession code SRP040582 . The H. oligactis transcriptome assembly has been deposited under BioSample code SAMN02700548, accession code GBFD00000000 in the NCBI TSA database, and is also available from http://www.compagen.org . The microarray custom design and raw data have been deposited in the NCBI Gene Expression Omnibus repository under the accession code GSE56287 . How to cite this article : Domazet-Lošo, T. et al. Naturally occurring tumours in the basal metazoan Hydra . Nat. Commun. 5:4222 doi: 10.1038/ncomms5222 (2014).